Aromatic C-H addition of ketones to imines enabled by manganese catalysis Selectivity control of varied C–H bonds in a complex molecule is a long-standing goal and still a great challenge in C–H activation field. Most often, such selectivity is achieved by the innate reactivity of different C–H bonds. In this context, the classic Mannich reaction of acetophenone derivatives and imines is ascribed to the more reactive C(sp 3 )–H bonds α to the carbonyl, with the much less reactive aromatic C(sp 2 )–H bonds remaining intact. Herein we report an aromatic C(sp 2 )–H addition of ketones to imines enabled by manganese catalysis, which totally reverses the innate reactivity of C–H bonds α to the carbonyl and those on the aromatic ring. Diverse products of ortho -C–H aminoalkylated ketones, cyclized exo -olefinic isoindolines, and three-component methylated isoindolines can be successfully accessed under mild reaction conditions, which significantly expands the synthetic utilities of ketones as simple bulk chemicals. Ketones such as acetophenone are considered among the most easily accessible and practically useful building blocks in both laboratories and chemical industries. They undergo various transformations on the α-C–H bonds with a wide range of electrophiles, which now constitute an important chapter in many textbooks of organic chemistry. Among them, the Mannich reaction, enabling an addition of the α-C–H bond to an iminium ion or imine, has been known for a long time and represents one of the most classic reactions of ketones (Fig. 1 a) [1] , [2] , [3] . It proceeds easily under either acidic or basic reaction conditions to afford the β-amino carbonyl and/or other derivatives. Of note, the C(sp 2 )–H bonds ortho to the carbonyl of ketones remain intact during this process, which shows that the reactivity of α-C–H bonds holds an absolute superiority over that of the ortho -C–H bonds on the benzene ring. Fig. 1 Innate and reversed reactivity of C–H bonds in ketones with imines. a The classic Mannich reaction of innately reactive α-C(sp 3 )–H bonds. b Mn-catalyzed ortho -C(sp 2 )–H addition by reversing the reactivity of C–H bonds (this work) Full size image Recently, the directed C–H transformations of ketones [4] , [5] have attracted immense attentions due to the prevalence of the carbonyl group in natural products, pharmaceuticals, and organic synthesis. Since the pioneering work of Ru-catalyzed aromatic C–H alkylation by Murai and others [6] , [7] , [8] , [9] , [10] , the ketone-directed C–H alkenylation [11] , [12] , [13] , arylation [14] , [15] , [16] , and amination [17] , [18] , [19] , among others [20] , [21] , [22] , [23] , [24] , [25] have been elegantly demonstrated. Note that in most of these protocols the undesirable reactions on α-C–H bonds of ketones are not notorious by choosing suitable reaction partners. Moreover, these reactions have heavily relied on late transition metals (Ru, Rh, Pd, and Ir) so far. Developments of earth-abundant base metal catalyzed site-selective aromatic C–H transformations of ketones with more challenging imine electrophiles have not been reported yet. Despite of their huge synthetic interests, considerable challenges still remain in these processes, such as the formidably competitive Mannich and/or Aldol-type reactions of α-C–H bonds of ketones, the relatively inert reactivity of aromatic C–H bonds with a weakly coordinating ketone group [26] , and the lower catalytic reactivity of base metals compared with the precious ones. To address these issues, we resort to manganese-promoted C–H activation [27] , [28] , [29] , [30] , [31] , [32] , [33] , [34] , [35] , [36] , [37] , [38] , [39] , [40] , [41] , [42] , [43] , in which the stoichiometric cyclomanganation of ketones was shown by Kaesz and Nicholson as early as in 1975 [44] , [45] . However, the manganese-catalyzed aromatic C–H transformations of ketones remain elusive. Here, we describe, as our continuous interest in manganese catalysis [31] , [32] , [33] , [34] , [35] , [36] , a manganese-catalyzed site-selective aromatic C–H addition of ketones to imines under mild reaction conditions, while the conventional Mannich reaction is completely suppressed. Moreover, cyclized exo -olefinic isoindoline and three-component methylated isoindoline derivatives can be selectively obtained. Thus, such diverse reactivity provides a straightforward and efficient way to access varied functionalized isoindolines from simple ketones and imines. Optimization of Reaction conditions As shown in Fig. 1b , we intended to develop a manganese-catalyzed aromatic C–H addition of ketones to imines. 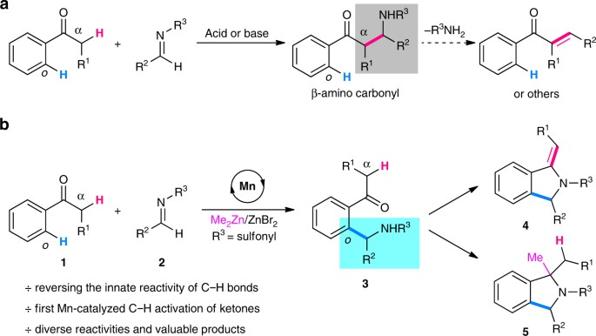Fig. 1 Innate and reversed reactivity of C–H bonds in ketones with imines.aThe classic Mannich reaction of innately reactive α-C(sp3)–H bonds.bMn-catalyzedortho-C(sp2)–H addition by reversing the reactivity of C–H bonds (this work) At the outset, in order to simplify the reaction outcome we chose t -butyl phenyl ketone 1a and imine 2a as model substrates to screen the reaction parameters (see Supplementary Table 1 for more details). The optimal reaction conditions were obtained by using MnBr(CO) 5 as a catalyst, Me 2 Zn/ZnBr 2 as promoters in the solvent of 1,2-dichloroethane (DCE) at 60 °C. We then evaluated the reaction chemoselectivity by using acetophenone 1v bearing α-C–H bonds as a substrate which was commonly used in the Mannich reaction (Fig. 2 ). Interestingly, when the reaction was carried out in the absence of MnBr(CO) 5 , the Mannich reaction took place overwhelmingly followed by elimination of an amine of the β-amino carbonyl intermediate to afford chalcone 6 in 46% gas chromatography–mass spectrometry (GC-MS) yield. In a sharp contrast, under the manganese catalysis product 4a resulting from aromatic C–H addition/cyclization/elimination was obtained in 66% isolated yield. Remarkably, this represents a reversal of the usual reactivity between ortho C(sp 2 )–H bonds and α-C(sp 3 )–H bonds of ketones with imines achieved by using a transition metal catalyst. Fig. 2 Evaluating the C–H bond selectivity of ketones by manganese-based catalytic system. a GC-MS yield. b Isolated yield. DCM dichloromethane, ND not detected Full size image Investigations on substrate scopes With the optimized conditions in hand, the scope of ketones was first explored (Fig. 3 ). Aromatic ketones bearing a wide range of electronically varied functional groups on the benzene ring delivered the corresponding aromatic C–H addition products successfully ( 3a–j ). Ketones containing two sterically biased C–H bonds reacted with imine 2a at the less hindered positions exclusively giving products 3k and 3l respectively. Heteroaromatic ketone 2,2-dimethyl-1-(thiophen-2-yl)propan-1-one 1m was also a viable substrate affording the expected product 3m in synthetically useful yield. Replacing the t -butyl group of 1a by other alkyl groups bearing α-C–H bonds, the reaction worked as well even at room temperature or 40 °C leading to the expected products smoothly ( 3n–p ). Of note, no Mannich-type products were detected in these reactions and the carbonyl-remaining products provide a handle for further synthetic elaborations. Importantly, benzophenone 1q and phenyl( o -tolyl)methanone 1r were also suitable substrates giving the mono -C–H addition products in good yields ( 3q , 3r ). In addition, arenes and heteroarenes bearing nitrogen-containing directing groups could also undergo the corresponding C–H aminoalkylation reaction with the current reaction conditions ( 3s–u ). [46] , [47] , [48] , [49] , [50] , [51] Of note, Ackermann has elegantly disclosed the related C–H aminoalkylation of indoles with imines in the absence of zinc additives at higher tempreture. [40] Fig. 3 Scope of ketones for the mono -C–H addition reaction. Reaction conditions: 1 (1.5 mmol), 2a (0.5 mmol), MnBr(CO) 5 (0.05 mmol), Me 2 Zn (0.75 mmol, 1.2 M in toluene), ZnBr 2 (0.5 mmol), DCE (0.4 M), 60 °C, 10 h. a 1n (2.0 mmol), DCM (0.1 M), r.t., 16 h. b 1o (2.0 mmol), DCM (0.1 M), r.t., 1 h. c 1p (2.0 mmol), DCM (0.1 M), 40 °C, 1 h. DCE 1,2-dichloroethane, DCM dichloromethane Full size image Next, the scope of imines was surveyed with ketone 1a as the model substrate (Fig. 4 ). Both electron-donating and electron-withdrawing groups were well tolerated in the reaction with the former ones giving relatively higher yields of the aromatic C–H addition products ( 3v-A ). Ortho- and meta- substituents on the benzene ring of imines showed comparable effect on the reaction yields ( 3v vs. 3B , 3C ). Naphthyl imines with extended conjugation delivered the expected products smoothly ( 3D , 3E ). It seemed that the steric hindrance had limited influence on the reaction outcome ( 3B , 3D ). Heteroaromatic imine and p -tolylsulfonyl imine were also amenable to this protocol ( 3F , 3G ). 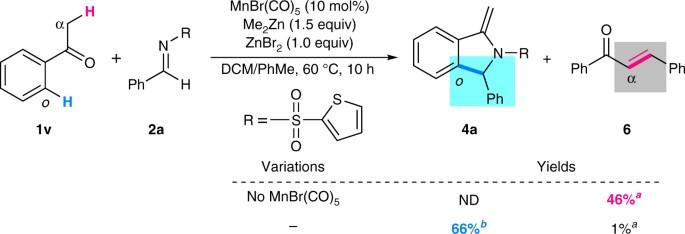Fig. 2 Evaluating the C–H bond selectivity of ketones by manganese-based catalytic system.aGC-MS yield.bIsolated yield.DCMdichloromethane,NDnot detected Unfortunately, aliphatic imines failed to afford the corresponding products under the reaction conditions. Fig. 4 Scope of imines for the mono -C–H addition reaction. Reaction conditions: 1a (1.5 mmol), 2 (0.5 mmol), MnBr(CO) 5 (0.05 mmol), Me 2 Zn (0.75 mmol, 1.2 M in toluene), ZnBr 2 (0.5 mmol), DCE (0.4 M), 60 °C, 10 h. DCE 1,2-dichloroethane Full size image When a chiral ketone, 1C of 96% ee, was used as a substrate and treated with imine 2a under the similar reaction conditions, the corresponding ortho -aminoalkylated product 3H was isolated in 66% yield with a dr value of 9.4:1 (Fig. 5 ). The major diastereo-isomer of 3H was in 96% ee, which reflected the ee value of ketone 1C . Furthermore, the structural configuration of the major diastereo-isomer was confirmed by single-crystal X-ray diffraction analysis. Fig. 5 A diastereoselective mono -C–H addition reaction using chiral ketone 1 C . a The major diastereo-isomer was shown. b Combined isolated yield. c Determined by 1 H NMR analysis of the crude product. DCM dichloromethane Full size image Interestingly, the exo -olefinic isoindoline products 4 could be selectively obtained from the reactions of imines and aryl alkyl ketones bearing α-C–H bonds by slightly tuning the reaction conditions (Fig. 6 ). Specifically, acetophenone 1v was treated with imine 2a at 60 °C for 2 h under the otherwise same conditions giving exo -olefinic isoindoline 4a in 66% isolated yield. The structure of 4a was unambiguously confirmed by single-crystal X-ray diffraction analysis. Introducing a methyl group into the para , meta , or ortho position of acetophenone resulted in the formation of the expected products successfully ( 4b–d ). Remarkably, the reaction of propiophenone with imine 2a provided exclusively isoindoline 4e with an E -configuration of the exo -cyclic C = C bond, which was again unambiguously confirmed by single-crystal X-ray diffraction analysis. The steric compulsion between the methyl group and (2-thienyl)sulfonyl group might account for the observed configuration of the double bond. 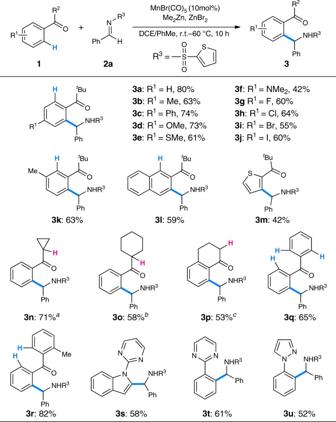Fig. 3 Scope of ketones for themono-C–H addition reaction. Reaction conditions:1(1.5 mmol),2a(0.5 mmol), MnBr(CO)5(0.05 mmol), Me2Zn (0.75 mmol, 1.2 M in toluene), ZnBr2(0.5 mmol), DCE (0.4 M), 60 °C, 10 h.a1n(2.0 mmol), DCM (0.1 M), r.t., 16 h.b1o(2.0 mmol), DCM (0.1 M), r.t., 1 h.c1p(2.0 mmol), DCM (0.1 M), 40 °C, 1 h.DCE1,2-dichloroethane,DCMdichloromethane 1-Tetralone and 1-benzosuberone were also proved to be suitable substrates affording the corresponding tricyclic products successfully under the slightly modified reaction conditions ( 4f , 4g ). A series of imines bearing electronically varied functional groups were applicable to this reaction leading to the expected exo -olefinic isoindoline products smoothly ( 4h–l ). p -Tolylsulfonyl imine was again susceptible to the reaction conditions giving the corresponding product in comparable yield ( 4m ). Fig. 6 Substrate scope for the [3 + 2] annulations giving exo -olefinic isoindolines 4 . Reaction conditions: 1 (2.0 mmol), 2 (0.5 mmol), MnBr(CO) 5 (0.05 mmol), Me 2 Zn (0.75 mmol, 1.2 M in toluene), ZnBr 2 (0.5 mmol), DCM (0.1 M), 60 °C, 2 h. a Combined yield of two regioisomers (3.9/1), major isomer 4c was shown. b Me 2 Zn (2.0 equiv. ), 100 °C, 10 h. DCM dichloromethane Full size image During our further investigations on the reaction parameters, we surprisingly found that a three-component reaction of ketone, imine, and dimethylzinc could be achieved simply by utilizing two equivalents of dimethylzinc at an elevated temperature under the otherwise same conditions (Fig. 7 ). Thus, a range of isoindolines bearing a tetra -substituted carbon center could be easily accessed from simple ketones and imines with moderate to good diastereoselectivity ( 5a–g ). The structures of the major cis -diastereoisomers 5c and 5d were both confirmed by single-crystal X-ray diffraction analysis. It should be noted that the use of t -butyl phenyl ketone 1a could not afford the corresponding three-component product presumably due to the increased steric hindrance of the congested tetra -substituted carbon center. Fig. 7 Substrate scope for the three-component reaction giving isoindolines 5 . Reaction conditions: 1 (2.0 mmol), 2 (0.5 mmol), MnBr(CO) 5 (0.05 mmol), Me 2 Zn (2.0 mmol, 1.2 M in toluene), ZnBr 2 (0.5 mmol), DCM (0.1 M), 100 °C, 10 h. The ratio of diastereoisomers (dr) was shown in parentheses. DCM dichloromethane Full size image Mechanistic studies To clarify the possible reaction pathways, a range of mechanistic experiments were conducted. First, the stoichiometric reaction of ketone 1a with MnBr(CO) 5 was examined and no product was detected (Fig. 8a ). While no reaction occurred with the assistance of ZnBr 2 , the addition of Me 2 Zn to the reaction resulted in the formation of five-membered manganacycle Mn-I in 28% isolated yield. Also, enolizable acetophenone 1v could delivered the corresponding manganacycle Mn-I′ in comparable yield, whose structure was confirmed by single-crystal X-ray diffraction analysis. MnMe(CO) 5 , generated in situ from the transmetalation of MnBr(CO) 5 with Me 2 Zn, might play a critical role in the step of C–H bond cleavage [35] . Second, treatment of Mn-I with imine 2a afforded the C–H addition product 3a in 27% 1 H NMR yield (Fig. 8b ). The reaction yields could be further improved by adding either Me 2 Zn or ZnBr 2 . Finally, the reactions of ketone 1a and imine 2a using manganacycle Mn-I or MnMe(CO) 5 as a catalyst were examined and the corresponding product 3a was formed in 74 and 80% yield, respectively (Fig. 8c ). These results suggested that both the manganacycle Mn-I and MnMe(CO) 5 might be the key intermediates in the reaction. Fig. 8 Mechanistic experiments. a Isolation of key intermediates Mn-I and Mn-I′ . b Stoichiometric reactions of Mn-I and imine 2a . c Reactions using Mn-I and MnMe(CO) 5 as a catalyst. DCE 1,2-dichloroethane Full size image Furthermore, deuterium-labeling experiments were carried out in order to probe the nature of the C–H bond cleavage. First, tert -butyl(pentadeuteriophenyl)methone 1a- d 5 was prepared and then subjected to the reaction conditions (Fig. 9a ). No loss of deuterium was observed at the ortho positions of 1a- d 5 , which suggested an irreversible C–H bond cleavage step in the reaction. Next, two parallel reactions of 1a and 1a- d 5 with imine 2a respectively were conducted (Fig. 9b ). As a result, a kinetic isotope effect (KIE) value of 3.2 implied the C–H bond cleavage might be involved in the turnover-limiting step or in a prior step with a lower activation barrier [52] . Fig. 9 Deuterium-labeling experiments. a Probing the reversibility of the C–H bond cleavage. b Probing the kinetic isotope effect. DCE 1,2-dichloroethane Full size image Based on the above results and literature clues [35] , [43] , [53] , a plausible reaction mechanism was depicted in Fig. 10 . The reaction starts with the formation of MnMe(CO) 5 from MnBr(CO) 5 and Me 2 Zn. It further reacts with ketone 1 to give five-membered manganacycle Mn-I followed by addition to imine 2 yielding seven-membered manganacycle Mn-II . Transmetalation of Mn-II with Me 2 Zn affords intermediate Mn-III , which undergoes a ligand exchange with substrate 1 to produce species Mn-IV and Zn-I . An intramolecular C–H activation occurs in Mn-IV regenerating Mn-I and releasing methane [35] . 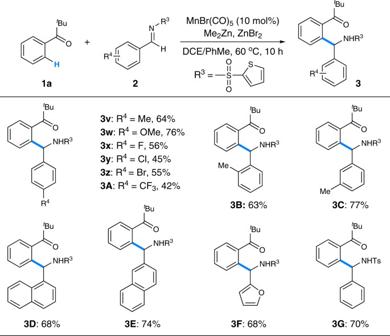Fig. 4 Scope of imines for themono-C–H addition reaction. Reaction conditions:1a(1.5 mmol),2(0.5 mmol), MnBr(CO)5(0.05 mmol), Me2Zn (0.75 mmol, 1.2 M in toluene), ZnBr2(0.5 mmol),DCE(0.4 M), 60 °C, 10 h.DCE1,2-dichloroethane Hydrolysis of Zn-I gives product 3 . Meanwhile, Zn-I may also undergo an intramolecular cyclization to yield intermediate Zn-II , which is followed by either an elimination of zinc salt giving exo -olefinic isoindoline 4 or an intermolecular nucleophilic substitution with Me 2 Zn forming isoindoline 5 under well-controlled reaction conditions. Fig. 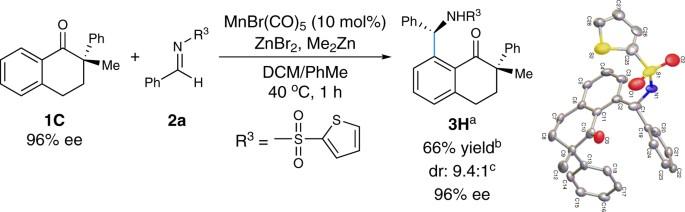Fig. 5 A diastereoselectivemono-C–H addition reaction using chiral ketone1 C.aThe major diastereo-isomer was shown.bCombined isolated yield.cDetermined by1H NMR analysis of the crude product.DCMdichloromethane 10 A proposed reaction mechanism. Key steps include formation of Mn-I followed by addition to imine yielding Mn-II , transmetalation of Mn-II with Me 2 Zn giving Mn-III , then producing Mn-IV and Zn-I by a ligand exchange with 1 , and C–H activation of Mn-IV regenerating Mn-I . Intramolecular cyclization of Zn-I yields Zn-II followed by either an elimination giving 4 or an intermolecular nucleophilic substitution with Me 2 Zn forming 5 Full size image In conclusion, aromatic C–H addition of ketones to imines was developed via manganese catalysis, which enabled to reverse the reactivity of labile C(sp 3 )–H bonds α to the carbonyl and inert C(sp 2 )–H bonds on the benzene ring of ketones. Thus, the classic Mannich reaction was completely depressed and a series of valuable products, namely the ortho -C–H aminoalkylated ketones, cyclized exo -olefinic isoindolines, and three-component methylated isoindolines, can be selectively achieved. Meanwhile, this protocol also represents a manganese-catalyzed aromatic C–H bond transformation of ketones since the parent stoichiometric cyclomanganation reaction was reported in 1975 [44] , [45] . Further explorations on the manganese-catalyzed C–H activation reactions of ketones are underway in our laboratory. General procedure for the formation of products 3 To a 25 ml flame-dried Schlenk tube was added ZnBr 2 (0.5 mmol, 112.5 mg, stored in glove box), MnBr(CO) 5 (0.05 mmol, 10.0 mol%, 13.8 mg), DCE (1.25 mL), 2,2-dimethyl-1-phenylpropan-1-one 1a (1.5 mmol, 243.0 mg), ( E )- N -benzylidenethiophene-2-sulfonamide 2a (0.5 mmol, 125.5 mg), and Me 2 Zn (0.75 mmol, 1.2 M in toluene, 0.625 mL) sequentially under nitrogen. The tube was sealed and stirred at 60 °C for 10 h. After completion, the reaction mixture was diluted with ethyl acetate (5.0 mL) and filtered through a short pad silica gel washing with ethyl acetate (20 mL). The filtrate was concentrated and purified by silica gel column chromatography to provide the product 3a in 80% yield. General procedure for the formation of products 4 To a Schlenk tube was added ZnBr 2 (0.5 mmol, 112.5 mg), MnBr(CO) 5 (0.05 mmol, 10.0 mol%, 13.8 mg), DCM (5.0 mL), acetophenone 1v (2.0 mmol, 240.0 mg), ( E )- N -benzylidene thiophene-2-sulfonamide 2a (0.5 mmol, 125.5 mg), and Me 2 Zn (0.75 mmol, 1.2 M in toluene, 0.625 mL) sequentially under nitrogen. The tube was sealed and stirred at 60 °C for 2 h. After completion, the reaction mixture was diluted with ethyl acetate (10 mL) and filtered through a short pad silica gel washing with ethyl acetate (20 mL). The filtrate was concentrated and purified by silica gel column chromatography to provide 4a in 66% yield. General procedure for the formation of products 5 To a Schlenk tube was added ZnBr 2 (0.5 mmol, 112.5 mg), MnBr(CO) 5 (0.05 mmol, 10.0 mol%, 13.8 mg), DCM (5.0 mL), propiophenone 1z (2.0 mmol, 276.0 mg), ( E )- N -benzylidenethiophene-2 -sulfonamide 2a (0.5 mmol, 125.5 mg), and Me 2 Zn (1.0 mmol, 1.2 M in toluene, 0.83 mL) sequentially under nitrogen. The tube was sealed and stirred at 100 °C for 10 h. After completion, the reaction mixture was diluted with ethyl acetate (10 mL) and filtered through a short pad silica gel washing with ethyl acetate (20 mL). The filtrate was concentrated and purified by silica gel column chromatography to provide 5a in 63% yield (dr = 3.1:1). 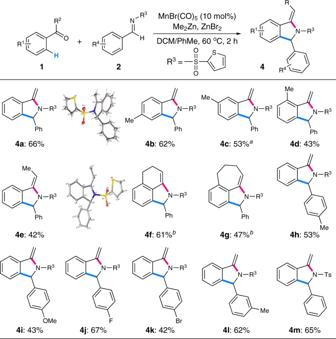Fig. 6 Substrate scope for the [3 + 2] annulations givingexo-olefinic isoindolines4. Reaction conditions:1(2.0 mmol),2(0.5 mmol), MnBr(CO)5(0.05 mmol), Me2Zn (0.75 mmol, 1.2 M in toluene), ZnBr2(0.5 mmol), DCM (0.1 M), 60 °C, 2 h.aCombined yield of two regioisomers (3.9/1), major isomer4cwas shown.bMe2Zn (2.0 equiv.), 100 °C, 10 h.DCMdichloromethane Data availability All data supporting the findings of this study are available within the article and its Supplementary Information file or from the authors on reasonable request. Supplementary crystallographic information files, which include structure factors, have been deposited with the Cambridge Crystallographic Data Centre (CCDC) as deposition numbers CCDC 1563929, 3H ; CCDC: 1532722, 4a ; CCDC: 1532723, 4e ; CCDC: 1532725, 5c ; CCDC: 1532724, 5d ; CCDC 1563930, Mn-I′ . 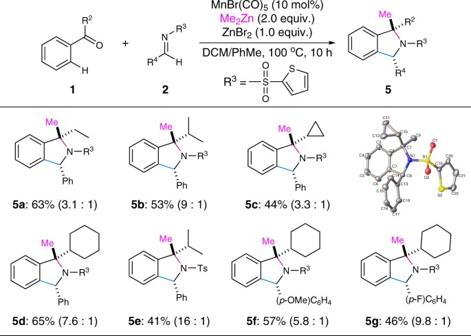Fig. 7 Substrate scope for the three-component reaction giving isoindolines5. Reaction conditions:1(2.0 mmol),2(0.5 mmol), MnBr(CO)5(0.05 mmol), Me2Zn (2.0 mmol, 1.2 M in toluene), ZnBr2(0.5 mmol), DCM (0.1 M), 100 °C, 10 h. The ratio of diastereoisomers (dr) was shown in parentheses.DCMdichloromethane 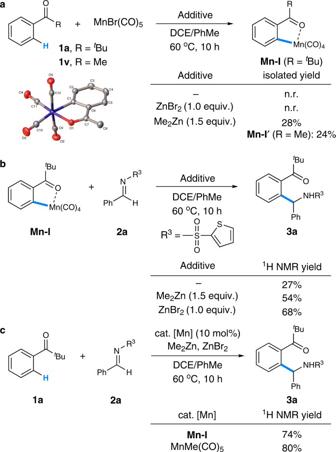Fig. 8 Mechanistic experiments.aIsolation of key intermediatesMn-IandMn-I′.bStoichiometric reactions ofMn-Iand imine2a.cReactions usingMn-Iand MnMe(CO)5as a catalyst.DCE1,2-dichloroethane 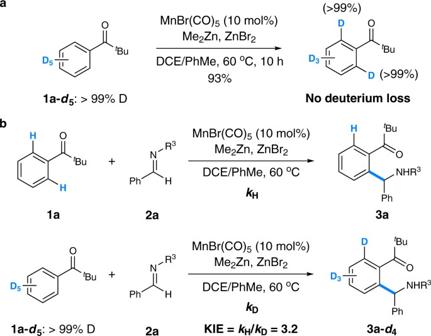Fig. 9 Deuterium-labeling experiments.aProbing the reversibility of the C–H bond cleavage.bProbing the kinetic isotope effect.DCE1,2-dichloroethane 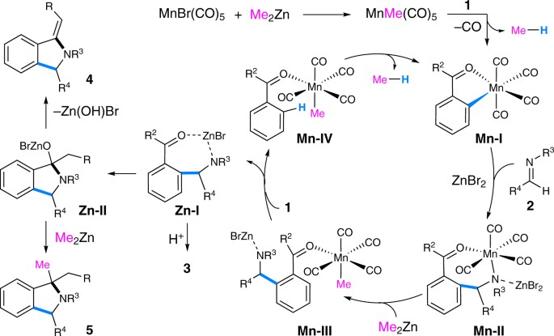Fig. 10 A proposed reaction mechanism. Key steps include formation ofMn-Ifollowed by addition to imine yieldingMn-II, transmetalation ofMn-IIwith Me2Zn givingMn-III, then producingMn-IVandZn-Iby a ligand exchange with1, and C–H activation ofMn-IVregeneratingMn-I. Intramolecular cyclization ofZn-IyieldsZn-IIfollowed by either an elimination giving4or an intermolecular nucleophilic substitution with Me2Zn forming5 These data files can be obtained free of charge from http://www.ccdc.cam.ac.uk/data_request/cif .